TwoFLXfamily members are non-redundantly required to establish the vernalization requirement inArabidopsis Studies of natural genetic variation for the vernalization requirement in Arabidopsis have revealed two genes, FRIGIDA and FLOWERING LOCUS C ( FLC ), that are determinants of the vernalization-requiring, winter-annual habit. In this study, we show that FLOWERING LOCUS C EXPRESSOR-LIKE 4 ( FLL4 ) is essential for upregulation of FLC in winter-annual Arabidopsis accessions and establishment of a vernalization requirement. FLL4 is part of the FLOWERING LOCUS C EXPRESSOR gene family and both are non-redundantly involved in flowering time control. Epistasis analysis among FRIGIDA , FLL4 , FLOWERING LOCUS C EXPRESSOR and autonomous-pathway genes reveals that FRIGIDA fve exhibits an extreme delay of flowering compared with fri fve , but mutants in other autonomous-pathway genes do not, indicating that FVE acts most antagonistically to FRIGIDA . FLL4 may represent a new member of a FRI-containing complex that activates FLC . A rabidopsis thaliana has been used as a model for studying flowering time regulation. Major environmental inputs that induce flowering in Arabidopsis and many other plant species are prolonged exposure to cold (vernalization) and photoperiod. There are two types of Arabidopsis accessions, summer-annual and winter-annual. Summer-annual accessions flower rapidly without vernalization, whereas winter-annual accessions require vernalization for rapid flowering [1] . Studies of natural genetic variation have revealed two genes, FRIGIDA ( FRI ) and FLOWERING LOCUS C ( FLC ), that are determinants of the winter-annual habit [2] , [3] . FLC encodes a MADS-box transcription factor that suppresses flowering [4] , and FRI encodes a nuclear protein containing coiled-coil domains [5] . FRI is essential for FLC expression to be sufficiently high to repress flowering in the fall [6] . During vernalization, FLC is repressed, resulting in plants that flower in the spring [4] , [7] . Summer-annual accessions typically contain naturally occurring mutations in FRI , resulting in attenuated FLC expression such that flowering occurs without vernalization [6] , [8] . In addition to FRI , a range of genes have been identified that are required for the elevated FLC expression that confers a winter-annual habit [9] . Some of these genes encode proteins involved generally in chromatin modification and RNA processing. Therefore, loss of these genes results in both a rapid-flowering phenotype due to loss of FLC activation and pleiotropic phenotypes due to misregulation of other genes. This class includes components of the RNA polymerase II-associated factor 1 complex ( VERNALIZATION INDEPENDENCE 3 , VERNALIZATION INDEPENDENCE 4 , EARLY FLOWERING 7 ( ELF7 ) and ELF8 ) (refs 10 , 11 , 12 ), a histone H3K36 methyltransferase ( ELF IN SHORT DAYS ( EFS ) [13] , histone H3K4 methyltransferases ( ARABIDOPSIS TRITHORAX-LIKE 1 ( ATX1 ), ATX2 and ATX-RELATED 7 ( ATXR7 )) (refs 14 , 15 ), a SWR1-related, nucleosome-remodeling factor ( PHOTOPERIOD INDEPENDENT EARLY 1 , ACTIN-RELATED PROTEIN 4 , SUPPRESSOR OF FRI 3 ( SUF3 )/ ACTIN-RELATED PROTEIN 6 / EARLY IN SHORT DAYS 1 (refs 16 , 17 , 18 , 19 ), RNA-processing factors ( SERRATE and HUA2 ) (refs 20 , 21 ) and a mRNA cap-binding protein ( ABA HYPERSENSITIVE 1 / CAP-BINDING PROTEIN 80 ) (ref. 22 ). In contrast to general regulators for which mutations have pleiotropic effects, mutations in other regulators of FLC affect only flowering and thus might be specific to the vernalization system. One example is FRI , which by genome-wide expression analyses affects only FLC expression [8] . Several mutations in other genes caused rapid flowering by attenuating FLC expression without pleiotropic effects [23] , [24] , [25] , [26] , [27] . A recent study indicates that the proteins encoded by all of these are members of a multimeric FRI complex [23] ; liquid chromatography-tandem mass spectrometry using 35S-myc:FRI identified FRI -LIKE 1 (FRL1), FRI ESSENTIAL 1 (FES1), SUF4 and FLC EXPRESSOR (FLX) [23] as associated with FRI. One of FRI complex components, FLX , is a member of a five-gene family containing FLX , FLX-LIKE 1 ( FLL1 ), FLL2 , FLL3 and FLL4 (ref. 23 ). Although only FLX was identified as a FRI complex component using liquid chromatography-tandem mass spectrometry, the other family members physically interact with FRI in yeast two-hybrid assay [23] . Furthermore, yeast one-hybrid assays indicated that FLX and FLL1 have transcriptional activity. However, it is not known whether other FLX family members have a role in activating FLC . In addition to the FLC activators discussed above, genetic screens have identified several vernalization-insensitive mutants, which encode FLC repressors that participate in the vernalization pathway such as VERNALIZATION-INSENSITIVE 3 ( VIN3 ), VERNALIZATION 1 ( VRN1 ), VRN2 and VIN3-LIKE 1 / VRN5 (refs 24 , 25 , 26 , 27 , 28 ). These genes are required to epigenetically silence FLC expression via enriching H3K9 and/or H3K27 methylation of FLC chromatin. VIN3 is specifically upregulated during cold exposure, and VIN3 expression is rapidly extinguished after plants are returned to warm conditions [24] . Here we report that a FLX family member, FLL4 , is essential for FLC upregulation in winter-annual accessions. Furthermore, we show that only two FLX family members, FLX and FLL4 , are non-redundantly involved in flowering time control. Finally, we show that some putative FRI complex components have a role in flowering time control in the absence of a FRI. Our findings reveal further molecular insight into the control of vernalization. Two suppressors alter VIN3 and FLC expression without cold Previous studies have reported the identification of mutants that suppress the delayed flowering that occurs in the absence of vernalization in the line Columbia (Col) FRI , which was generated by introgression of functional Sf-2 FRI allele [4] , [29] . We screened additional ethyl methane sulfonate-generated mutants in Col FRI for rapid flowering lines that exhibited two properties of vernalized Arabidopsis plants in the absence of cold exposure: reduced FLC expression and increased VIN3 expression. In wild type, VIN3 is expressed only after a relatively long period of cold exposure [24] . From 98 lines initially identified as rapid flowering, we found two independent mutants that exhibited both reduced FLC expression and increased VIN3 expression. These mutants, which we now refer to as flx-3 and flx-like 4-1 ( fll4-1 ) ( Fig. 1a ) were chosen for further study because they appeared identical to Col and vernalized Col FRI ( Fig. 1c )—that is, there were no apparent pleiotropic phenotypes and they exhibited features of vernalized plants in the absence of cold exposure. 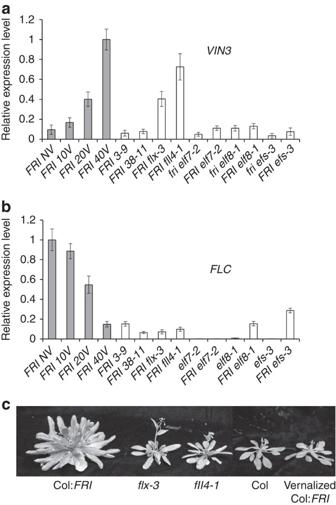Figure 1:flx-3andfll4-1alterVIN3andFLCexpression without cold. flx-3andfll4-1exhibitVIN3upregulation (a) andFLCdownregulation (b) without vernalization.FRI 3-9andFRI 38-11were selected as negative controls forVIN3expression from among theFRI-suppressor mutants we identified.FLCandVIN3expression were also monitored infri elf7-2,FRI elf7-2,fri elf8-1,FRI elf8-1,fri efs-3andFRI efs-3as additional controls. (c) Flowering phenotype offlx-3andfll4-1. All of the expression data are presented as mean values of three biological replicates. Error bars indicate s.d. Figure 1: flx-3 and fll4-1 alter VIN3 and FLC expression without cold. flx-3 and fll4-1 exhibit VIN3 upregulation ( a ) and FLC downregulation ( b ) without vernalization. FRI 3-9 and FRI 38-11 were selected as negative controls for VIN3 expression from among the FRI -suppressor mutants we identified. FLC and VIN3 expression were also monitored in fri elf7-2 , FRI elf7-2 , fri elf8-1 , FRI elf8-1 , fri efs-3 and FRI efs-3 as additional controls. ( c ) Flowering phenotype of flx-3 and fll4-1 . All of the expression data are presented as mean values of three biological replicates. Error bars indicate s.d. Full size image Mutations in FLL4 and FLX give rise to suppressor phenotypes To map the location of the genes responsible for the rapid-flowering phenotype of the two mutants that exhibited vernalization-independent increased VIN3 and decreased FLC expression, the mutants were crossed with a line in which FRI FLC had been introgressed into the Landsberg erecta genetic background [4] . The F1 generations exhibited delayed flowering, and in the F2 generations, delayed to rapid flowering clearly segregated in a 3:1 manner, indicating that in each line rapid flowering was a single-gene, recessive trait. The locations of the mutations were mapped in the F2 generations using a combination of simple sequence length polymorphism (SSLP) and derived cleaved amplified polymorphic sequence (dCAP) markers, which are polymorphic between Col-0 and Landsberg erecta [30] . One mutation was narrowed down to an interval between 24.78 and 24.91 MB on chromosome 5. Sequence analysis of this interval revealed a nonsense mutation in the first exon of AT5g61920 , FLL4 ( Supplementary Fig. S1a ). FLL4 had not previously been identified as being involved in flowering time control. The other mutation mapped on the lower arm of chromosome 2 around 12.09 MB. This region contained a gene known as FLX , which had previously been identified as a suppressor of FRI/FLC -mediated delayed flowering [23] , [31] . Further mapping and sequencing analysis identified that this suppressor line contained a single-base change in the first exon of AT2G30120 / FLX that resulted in the conversion of an arginine to a lysine residue at amino acid position 176 ( Supplementary Fig. S1b ). This arginine is conserved among all FLX family members ( Supplementary Fig. S2 ). To simultaneously evaluate whether the rapid-flowering phenotype of the mutants is indeed caused by mutations in FLL4 and FLX and whether there are any effects of overexpression, 35S-driven FLL4 and FLX were transformed into the respective mutant lines, and the phenotype was assessed. Introduction of 35S-driven FLL4 in fll4-1 and 35S-driven FLX in flx-3 rescued the mutant phenotype in all 12 lines examined for 35S::FLL4 and all 9 lines examined for 35S::FLX ( Fig. 2 ). Also, the flx suppressor was crossed to another flx allele (flx-2) that has been previously described [23] . The F1 plants retained the mutant phenotype indicating that we had identified another allele of FLX , which we designate as flx-3 ( Fig. 2 ). 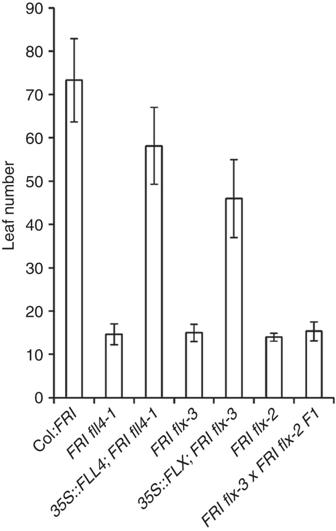Figure 2: The rapid-flowering phenotype results from lesions in bothFLL4andFLX. Flowering behaviour is represented by the number of rosette leaves formed on the primary stem before the transition to flowering of plants grown in long days without vernalization. Flowering was monitored in the transgenic lines to determine whetherFLL4andFLXcan rescue the flowering phenotype inFRI fll4andFRI flx. Flowering ofFRI flx-3×FRI flx-2F1 was also monitored. All of the flowering time data are presented as mean values of 12 individual plants except35S::FLX;FRI flx-3(nine individuals). Error bars indicate s.d. Figure 2: The rapid-flowering phenotype results from lesions in both FLL4 and FLX. Flowering behaviour is represented by the number of rosette leaves formed on the primary stem before the transition to flowering of plants grown in long days without vernalization. Flowering was monitored in the transgenic lines to determine whether FLL4 and FLX can rescue the flowering phenotype in FRI fll4 and FRI flx . Flowering of FRI flx-3 × FRI flx-2 F1 was also monitored. All of the flowering time data are presented as mean values of 12 individual plants except 35S::FLX ; FRI flx-3 (nine individuals). Error bars indicate s.d. Full size image Suppression of delayed flowering does not require VIN3 As discussed above, the fll4 and flx suppressors were chosen for further study because they exhibited both increased VIN3 expression, reduced FLC expression and rapid flowering in the absence of cold exposure. To determine whether the FLC suppression and rapid flowering of fll4 and flx is dependent on cold-independent VIN3 expression, we generated FRI fll4 vin3 , FRI flx vin3 and FRI fll4 flx vin3 and measured flowering time in these lines ( Fig. 3 ). There is no difference in the level of suppression of FRI FLC -mediated delayed flowering when VIN3 is present or absent in long days ( Fig. 3a ) or short days ( Fig. 3c ); thus, fll4 and flx suppression of FRI FLC -delayed flowering does not require VIN3 . 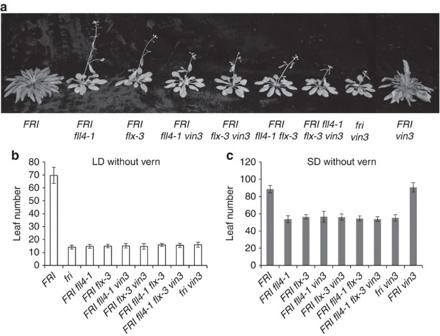Figure 3:VIN3is not required for the rapid flowering offll4andflx. The requirement forVIN3was evaluated by determining the flowering phenotype offll4andflxwith and withoutVIN3in long days (a,b) and short days (c). All of the flowering time data are presented as mean values of 12 individual plants. Error bars indicate s.d. Figure 3: VIN3 is not required for the rapid flowering of fll4 and flx. The requirement for VIN3 was evaluated by determining the flowering phenotype of fll4 and flx with and without VIN3 in long days ( a , b ) and short days ( c ). All of the flowering time data are presented as mean values of 12 individual plants. Error bars indicate s.d. Full size image Lesions in other FLX family members do not affect flowering The Arabidopsis genome contains five FLX family members. The FLX family is plant-specific and does not appear to share any motifs with other proteins. Among the five members, FLL4 and FLX proteins share 30% identity and 50% similarity. FLL1, FLL2 and FLL3 each have 38%, 26% and 29% identities, and 63%, 41% and 50% similarities with FLX, respectively ( Supplementary Fig. S2 ). To determine whether lesions in other FLX family members can suppress FRI -mediated delayed flowering similar to the suppression caused by fll4 and flx mutants, fll1 , fll2 and fll3 mutants were crossed with Col FRI , and from the resulting F2 generation, the flowering behaviour of homozygous mutants in the presence of FRI was determined. Mutations in these other FLX family members have no effect on flowering ( Supplementary Fig. S3 ) as also noted by Choi et al . [23] Thus, based on single mutant analysis, only two members, FLL4 and FLX , appear to be necessary for the winter-annual flowering habit. It is, however, possible that other family members have redundant function and that double mutants could have a flowering phenotype. FLL4 and FLX have non-redundant roles in flowering Because only FLX has transcriptional activity in a yeast one-hybrid assay, Choi et al . [23] speculated that FLX is the only protein among the five FLX family members involved in FRI/FLC -mediated flowering time control. However, Choi et al . [23] also showed that all FLX family members interact with FRI in a yeast two-hybrid assay. Our results clearly show that both FLL4 and FLX have a role in flowering time control. We took two approaches to determine whether the roles of FLL4 and FLX are redundant or non-redundant. First, we generated fll4 and flx double mutants in the FRI background. If both FLL4 and FLX contributed an identical dosage-dependent protein function (redundant roles), then a double mutant might be expected to flower earlier than the single mutants. However, flx-2/fll4-1 and flx-3/fll4-1 double mutants were identical with respect to flowering to the single mutants flx-2 or flx-3 and fll4-1 in the FRI background under both long days ( Fig. 4a ) and short days ( Fig. 4b ). In addition, the double mutants did not exhibit a further decrease of FLC expression ( Fig. 4c ). These data are consistent with non-redundant roles in for FLX and FLL4 in flowering time control. 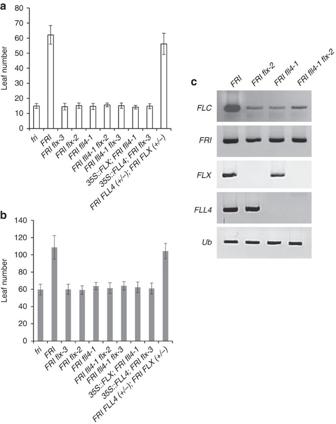Figure 4: Evaluation of redundancy betweenFLL4andFLX. (a) Flowering was monitored in two different versions of the double mutant,flx-2 fll4-1andflx-3 fll4-1, in the presence ofFRI, relative to each single mutant; the effects ofFLXoverexpression in thefll4mutant andFLL4overexpression in theflxmutant were also determined in long days (a) and short days (b) without vernalization. (c) Transcript levels ofFLC,FRI,FLXandFLL4in the mutant backgrounds were determined. All of the flowering time data are presented as mean values of 12 individual plants. Error bars indicate s.d. Figure 4: Evaluation of redundancy between FLL4 and FLX. ( a ) Flowering was monitored in two different versions of the double mutant, flx-2 fll4-1 and flx-3 fll4-1 , in the presence of FRI , relative to each single mutant; the effects of FLX overexpression in the fll4 mutant and FLL4 overexpression in the flx mutant were also determined in long days ( a ) and short days ( b ) without vernalization. ( c ) Transcript levels of FLC , FRI , FLX and FLL4 in the mutant backgrounds were determined. All of the flowering time data are presented as mean values of 12 individual plants. Error bars indicate s.d. Full size image The double mutant analyses, however, cannot rule out a model in which FLL4 and FLX do have redundant roles, but that single mutants drop below the threshold of activity required for the FRI/FLC -mediated delay of flowering. In this case, a double heterozygote would be expected to behave like a homozygous single fll4 or flx mutant. However, the double heterozygote flx-3 FLX; fll4-1 FLL4 in the FRI background flowers identical to wild type under both long days ( Fig. 4a ) and short days ( Fig. 4b ) arguing against redundancy and a threshold model. A second approach to address the question of possible redundancy is to overexpress FLL4 in the flx background and to overexpress FLX in the fll4 background; overexpression of one gene rescuing the mutant phenotype of the other would be consistent with redundancy. Overexpression of FLL4 in flx-3 and overexpression of FLX in fll4-1 did not rescue the mutant phenotype in long days ( Fig. 4a ) and short days ( Fig. 4b ). The overexpression constructs are functional because the FLL4 overexpression construct rescues the fll4-1 mutant and the FLX overexpression construct rescues the flx-3 mutant ( Fig. 2 ). No additive phenotype of fll4 and flx with fri and frl1 We previously reported that a FRI family member, FRL1 , has a non-redundant role with FRI in the establishment of the winter-annual habit [32] . When either gene is mutated, the winter-annual habit is lost because FLC expression is attenuated. To evaluate whether there is an additive flowering phenotype in the fri and frl1 , and fll4 and flx mutants, the phenotype of fri FRL1 fll4 , fri FRL1 flx , FRI frl1 fll4 , FRI frl flx and fri FRL1 fll4 flx was assessed in long and short days ( Fig. 5a ). The flowering time of the mutants tested did not show additive flowering suppression relative to the single FRI -complex component mutants. These data are consistent with FLL4, FLX, FRI and FRL1, all having critical non-redundant roles in the FRI complex. 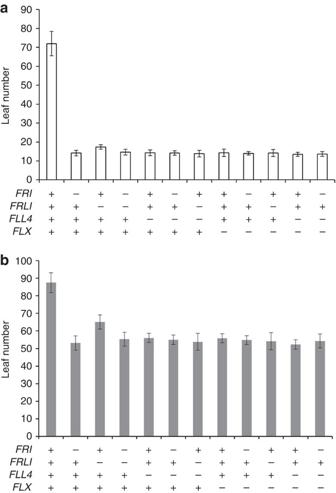Figure 5: Flowering phenotype of double and triple mutants. Flowering of the indicated mutant combinations was evaluated in long days (a) and short days (b) without vernalization. All of the flowering time data are presented as mean values of 12 individual plants. Error bars indicate s.d. Figure 5: Flowering phenotype of double and triple mutants. Flowering of the indicated mutant combinations was evaluated in long days ( a ) and short days ( b ) without vernalization. All of the flowering time data are presented as mean values of 12 individual plants. Error bars indicate s.d. Full size image fll4 and flx suppress the delayed flowering of fve and ld Andersson et al . [31] reported FLX as a flowering regulator based on the mutant phenotype in the C24 accession. A T-DNA-knockout mutant, flx-1 , repressed FLC expression, resulting in plants that flower earlier than C24 wild type. In this study, it was reported that FLX was not necessary for FLC activation when certain autonomous-pathway genes were downregulated. Furthermore, because FLX is part of the FRI complex [23] , and FRI is not required for the delayed flowering phenotype of autonomous-pathway mutants, it might be expected that loss of FLX or FLL4 would not affect the phenotype of autonomous-pathway mutants. We determined whether fll4 or flx mutations could suppress the delayed flowering that results from loss of function of autonomous-pathway genes, FPA [33] , FCA [34] , [35] , FLOWERING LOCUS D ( FLD ) [36] , [37] , LUMINIDEPENDENS ( LD ) [3] and FVE [38] . Accordingly double mutants were made between fpa-3 , fca-9 , fld-3 , ld-1 and fve-4 , and flx-3 and fll4-1 . The delayed flowering of autonomous-pathway mutants fpa , fca and fld was not suppressed by mutation of either fll4 or flx ( Fig. 6a ). However, the delayed flowering of ld and fve was suppressed by fll4 and flx mutations ( Fig. 6a ). The ld suppression was partial (compare fri,ld and flx or fri,ld and fll4 with fri alone), but the fve suppression was almost complete. FLC expression of the mutant lines was also monitored to determine if the flowering phenotype is a result of reduced FLC expression. As shown in Fig. 6b , loss of FLL4 and FLX suppresses delayed flowering of ld and fve via attenuating FLC expression ( Fig. 6b ). A suppression of the delayed flowering and FLC mRNA levels in ld and fve also results from lesions in SUF4 (ref. 39 ). 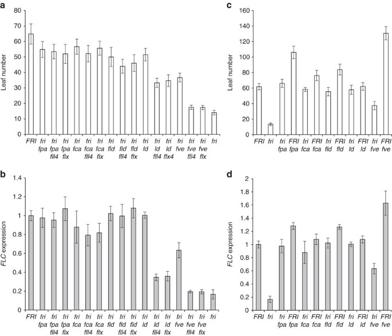Figure 6: The flowering time andFLCexpression phenotypes offll4andflxcombined with other flowering mutants. (a) Flowering offll4andflxmutants in autonomous mutantsfpa,fca,fld,ldandfvein long days without vernalization. (b) Transcript levels ofFLCin the genotypes froma. (c) Flowering of certain autonomous mutants with or withoutFRI. (d) Transcript levels ofFLCin the corresponding genotypes fromc. All flowering time data are presented as mean values of 12 individual plants, and all of the expression data are presented as mean values of three biological replicates. Error bars indicate s.d. Figure 6: The flowering time and FLC expression phenotypes of fll4 and flx combined with other flowering mutants. ( a ) Flowering of fll4 and flx mutants in autonomous mutants fpa , fca , fld , ld and fve in long days without vernalization. ( b ) Transcript levels of FLC in the genotypes from a . ( c ) Flowering of certain autonomous mutants with or without FRI . ( d ) Transcript levels of FLC in the corresponding genotypes from c . All flowering time data are presented as mean values of 12 individual plants, and all of the expression data are presented as mean values of three biological replicates. Error bars indicate s.d. Full size image We further tested whether loss of other FRI complex components can suppress the delayed flowering of fve . Interestingly, loss of FRL1, FES1 and SUF4 also caused a strong suppression of the delayed flowering of fve ( Supplementary Fig. S4 ). Antagonistic roles of FRI and FVE To explore the relationship between FVE and the FRI complex, we compared the flowering time of fve and certain other autonomous-pathway mutants with or without FRI . Interestingly, FRI fve exhibits a more extreme delay of flowering compared with fri fve , whereas other autonomous-pathway mutants fld , ld , fca and fpa did not exhibit such a large difference with or without FRI ( Fig. 6c ). The flowering time of autonomous mutants with or without FRI was also correlated with their FLC expression level ( Fig. 6d ). These data are consistent with a model in which FRI and FVE are acting oppositely on a similar molecular aspect of FLC regulation. FVE is thought to act by reducing the levels of histone acetylation [38] , [40] , which would attenuate FLC expression. FRI increases the levels of FLC histone modifications that promote active chromatin [13] , [23] . Thus, the opposing activities of FRI and FVE may be at the level of chromatin modification at the FLC locus. In the absence of FVE function, FRI activity might result in a ‘hyperactivated’ chromatin state at FLC , which is reflected in strongly delayed flowering and increased FLC mRNA levels. In a FRI background, loss of one of many putative FRI components is sufficient to reduce FLC expression to levels as low as those in rapid-cycling wild types that lack FRI [32] , [39] , [41] . As discussed above, however, loss of FVE provides a ‘sensitized’ background in which FRI causes a stronger delay in flowering. To further explore the roles of FLL4 and FLX in this sensitized background, we made double, triple and quadruple mutants among fri , fve , fll4 and flx . First, we compared the flowering behaviour of fve fll4 , fve flx and fve fll4 flx with or without FRI . The flowering of FRI fve fll4 and FRI fve flx was delayed compared with fri fve fll4 and fri fve flx ( Fig. 7a ). Thus, in the sensitized fve background, FRI causes a modest delay of flowering, in the absence of FLL4 or FLX . We also investigated the effect of these genetic combinations on FLC expression. The flowering behaviours were clearly correlated with FLC expression ( Fig. 7b ). These data indicate that the ability of FRI to delay flowering in the absence of FLL4 or FLX is mediated via FLC expression. 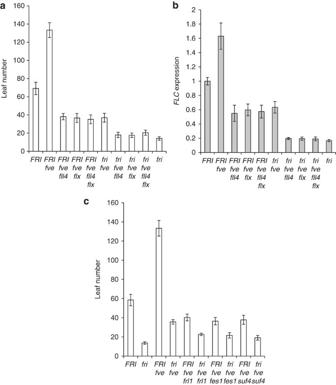Figure 7: Effect of loss of variousFRIcomplex components in thefvebackground. (a) Flowering was evaluated in various mutant combinations offri,fll4,flxandfvein long days without vernalization. (b) Transcript levels ofFLCin the genotypes studied froma. (c) The flowering phenotype ofFRIin various FRI complex component mutant backgrounds. All flowering time data are presented as mean values of 12 individual plants, and all of the expression data are presented as mean values of three biological replicates. Error bars indicate s.d. Figure 7: Effect of loss of various FRI complex components in the fve background. ( a ) Flowering was evaluated in various mutant combinations of fri , fll4 , flx and fve in long days without vernalization. ( b ) Transcript levels of FLC in the genotypes studied from a . ( c ) The flowering phenotype of FRI in various FRI complex component mutant backgrounds. All flowering time data are presented as mean values of 12 individual plants, and all of the expression data are presented as mean values of three biological replicates. Error bars indicate s.d. Full size image We also investigated whether or not FRI has activity when other putative complex components are mutated in the fve background ( Fig. 7c ). The flowering time of FRI fve frl1 , FRI fve fes1 and FRI fve suf4 was further delayed compared with fri fve frl1 , fri fve fes1 and fri fve suf4 , respectively. Thus, as was the case with fll4 and flx , FRI can cause a modest delay of flowering in the absence of FES1 , FRL1 and SUF4 when FVE is lacking. Our results demonstrate that two FLX family members, FLL4 and FLX , have non-redundant roles in FLC activation and the establishment of a vernalization requirement. FLL4 and FLX appear to be in the same flowering ‘pathway’ because fll4 and flx single mutants fully suppress the delayed flowering of a FRI -containing winter-annual line, and the double mutant did not show any additional flowering time change compared with the single mutants ( Fig. 4a ). That FLL4 and FLX have non-redundant roles in flowering is supported by the following evidence. First, as noted above, the fll4 flx double mutant has a phenotype identical to the single mutants. If there were redundancy, then the double mutant would be expected to have a more severe phenotype than the single mutants unless both single and double mutants fell below a threshold level of activity required to delay flowering. However, there is no flowering phenotype in the double heterozygote, fll4-1 FLL4 ; flx-3 FLX , arguing against a threshold model. Further evidence that FLL4 and FLX have non-redundant roles is that overexpression of FLX does not rescue a fll4 mutant and overexpression of FLL4 does not rescue a flx mutant. A model that accounts for non-redundancy, but similar function, is that both FLL4 and FLX are non-redundant members of a protein complex. This model is consistent with the results of Choi et al . [23] who showed that FRI and FLX are part of a multisubunit complex (the FRI complex) that is involved in FLC upregulation. In a yeast two-hybrid assay, Choi et al . [23] showed that all FLX family members can interact with FRI. Our results indicate that a fully functional FRI complex requires both FLX and FLL4 . It is intriguing that studies of the molecular basis of the vernalization requirement in Arabidopsis reveal at least two examples of the involvement of non-redundant members of a gene family. Specifically, both FRI and the FRI family members FRL1 or FRL2 (refs 32 , 42 ) and, as shown in this study, both FLX and the FLX family member FLL4 are necessary to create a vernalization requirement. The FRI and FLX gene families are present in all sequenced plant genomes including tropical species that do not have a vernalization requirement, and vernalization systems appear to have evolved independently and relatively recently in different plant lineages as an adaptation to temperate climates [9] . Thus, vernalization was not likely to be the ancestral role of the founding members of these gene families. If the ancestral role of such genes involved multimerization, then gene duplication could permit an additional copy to encode a protein that continues to function in the multimer complex along with the original member, and this would permit a version of the complex to diverge such that the diverging complex could assume a new function, such as elevating FLC expression to create a vernalization requirement. Consistent with this evolutionary path to a vernalization requirement, FLX, FRI and FRL1 reside in the same FRI complex [23] , and it is likely that FLL4 will be found in this complex as well. There are some intriguing differences in phenotype when different autonomous-pathway mutants are combined with FRI . FRI fve exhibits an extreme delay of flowering compared with fri fve , but FRI fld , FRI ld , FRI fca and FRI fpa do not, and the flowering time of these genotypes correlates with their FLC expression ( Fig. 6a ). FVE is an Arabidopsis homolog of the human histone-binding proteins retinoblastoma-associated protein 46 and 48 . As a component of a histone deacetlyase complex, FVE has been shown to be involved in a vernalization-independent system of FLC repression [38] , [40] , [43] , [44] , [45] . Thus, perhaps the FRI complex and its components such as FLL4 and FLX act antagonistically to FVE by increasing histone acetylation at FLC . Antagonistic functions would account for the strong delay of flowering caused by FRI in the fve mutant. Interestingly, it has been reported that the product of the autonomous-pathway gene FLD is also part of an FVE-containing histone deacetlyase complex [43] , [44] , [45] . However, our result that FRI fld does not exhibit the enhanced delayed flowered exhibited in FRI fve indicates that FVE and FLD act in separate pathways. This is consistent with previous reports that FVE functions independently of FCA , FPA and FLD to repress FLC expression via various loss/gain of function mutant series [37] , [46] . It is also intriguing that, in the absence of FRI , fll4 and flx mutants strongly suppress the delayed flowering of fve and, to a lesser extent, ld , but loss of FLL4 and FLX does not have a strong suppressive effect on other autonomous-pathway mutants. This could indicate that FLL4 and FLX have a function that is independent of the FRI complex if the complex was completely non-function in the absence of any components. Alternatively, in a ‘sensitized’ fve mutant background, the FRI complex might have residual FLC -promoting activity in the absence of FRI, and loss of FLL4 or FLX would attenuate this residual activity. This residual activity of the FRI complex without FRI would be consistent with the evolutionary model, noted above, of FRI evolving a role of ‘hyperactivating’ FLC to create a vernalization requirement; for example, there may have been a precursor complex to the current FRI complex that had moderate FLC -promoting activity. An in vitro system to study the interaction of FRI complex components and FVE with FLC would be useful to investigate this model. Plant materials and growth conditions The wild-type Arabidopsis plants used in this study were either wild-type Col/fri or a FRI introgression line (Col FRI) [4] , [29] . Seeds were sown on petri-plates containing 2 mM MES at pH 5.7, 0.8% (w/v) Phytoblend agar (Caisson Lab, North Logan, UT) and 0.65 gl −1 Peter’s Excel 15-5-15 CalMag fertilizer. Plated seeds were not stratified, and plants were transferred to soil. Plants were grown in Metro-Mix 360 (SUN GRO Horticulture) and fertilized with Peters Excel CalMag (15-5-15) at regular intervals in short days (8 h lights/16 h dark), long days (16 h lights/8 h dark) or continuous light from cool-white fluorescent tubes (photosynthetic photon flux density approximately 60–70 μmol m –2 s –1 ). For vernalization experiments, seedlings on agar were incubated at 4 °C in short days and transferred to soil after cold exposure. Gene expression analysis Total RNA was isolated from seedlings using TRIZOL reagent (Invitrogen) according to the manufacturer’s instructions and treated with RQ1 RNase-Free DNase (Promega). DNA-free RNA was used to generate cDNA using qScript cDNA SuperMix (Quanta Biosciences). After preparation of cDNA, quantitative real-time PCR was performed using Applied Biosystems 7500 Fast Real-Time PCR System. Ubiquitin 10 was used as an internal control. All primers used are listed in Supplementary Table S1 . Gene sequences and mutants All sequence data in this article can be found in GenBank Nucleotide Core under the following accession numbers: AT4G00650 ( FRI ), AT5G10140 ( FLC ), AT5G57380 ( VIN3 ), At2g30120 ( FLX ), At3g14750 ( FLL1 ), At1g67170 ( FLL2 ), At1g55170 ( FLL3 ) and At5g61920 ( FLL4 ). The mutant lines described in this manuscript are: elf7-2 (ref. 15 ), elf8-1 (ref. 12 ), efs-3 (ref. 13 ), flx-2 (ref. 23 ), fll1-1 (SALK_139524), fll2-1 (CS822746), fll3-1 (SALK_002678), vin3 (ref. 24 ), frl1-1 (ref. 32 ), fpa-7 (ref. 47 ), fca-9 (ref. 22 ), fld-3 (ref. 48 ), ld-1 (ref. 49 ), fve-4 (ref. 47 ), fes1-1 (ref. 41 ) and suf4 (ref. 39 ). Constructs For 35S::FLL4 and 35S::FLX , the coding regions of FLL4 and FLX were amplified by PCR, cloned into D-TOPO entry vectors (Invitrogen) and then moved into pGWB502 vectors (kindly provided from Dr Tsuyoshi Nakagawa) using the Gateway cloning system (Invitrogen) [50] . All primers used are listed in Supplementary Table S1 . How to cite this article: Lee, J. et al . Two FLX family members are non-redundantly required to establish the vernalization requirement in Arabidopsis . Nat. Commun. 4:2186 doi: 10.1038/ncomms3186 (2013)